Carbon nanotube network-silicon oxide non-volatile switches The integration of carbon nanotubes with silicon is important for their incorporation into next-generation nano-electronics. Here we demonstrate a non-volatile switch that utilizes carbon nanotube networks to electrically contact a conductive nanocrystal silicon filament in silicon dioxide. We form this device by biasing a nanotube network until it physically breaks in vacuum, creating the conductive silicon filament connected across a small nano-gap. From Raman spectroscopy, we observe coalescence of nanotubes during breakdown, which stabilizes the system to form very small gaps in the network~15 nm. We report that carbon nanotubes themselves are involved in switching the device to a high resistive state. Calculations reveal that this switching event occurs at ~600 °C, the temperature associated with the oxidation of nanotubes. Therefore, we propose that, in switching to a resistive state, the nanotube oxidizes by extracting oxygen from the substrate. As mobile electronic devices become more prevalent in society, the need for compact and densely packed non-volatile memory (NVM) continues to grow. As flash memory fast approaches its scaling and power limits [1] , [2] , other promising NVM technologies are being developed. Among these, resistive random access memory (RRAM) [3] , [4] has gained popularity in industry because it utilizes materials that are in common use in semiconductor processing. These MIM memory cells operate by switching the insulator between a high-resistive state (HRS) and a low resistive state (LRS). Whereas the switching mechanism to the LRS is well understood as oxygen atoms being removed from the lattice to form a conductive filament bridging the electrodes, there is not a complete consensus on the switching mechanism to return the MIM device to its HRS [3] . It is known, however, that the type of metal used to contact the insulator may influence this switching mechanism [5] , [6] . Regarding the insulator, while it is typical to use some kind of metal oxide [7] , [8] , [9] (for example, AlO x , HfO x , TiO x ) in the MIM cell, recently it was discovered that even silicon oxide could be switched between a HRS and a LRS [10] , [11] , [12] . Recently, break-gaps formed in isolated carbon nanotubes (CNTs) [10] , [13] , [14] have been used to obtain planar-oriented NVM cells on the nanometer scale. These switches truly push the scaling limits of an individual device. Such aggressive scaling has also been shown to reduce the power consumption of NVM cells, as less energy is needed to switch a smaller volume of material. Making planar devices from CNTs also enable novel devices for transparent electronics. However, individually broken CNTs cannot be manufactured yet, because there is large variation in gap size created from this process [14] , [15] . It is also difficult to control the placement of many individual CNTs at a high packing density, even in crossbar geometries [16] , [17] . To overcome some of these problems, patterned CNT networks or graphene [12] , [18] can be used instead. In this paper we focus on solution-deposited CNT networks, and how using sp 2 hybridized carbon as contacts will improve the device performance of MIM switches. We use transport measurements together with Raman spectroscopy to investigate the physical mechanisms behind the formation of the initial break-gap and the switching behaviour of the CNT-Si-CNT device. We find that during the initial breakdown of the CNT network, nanotubes localized around the break-gap begin to coalesce to thermally stabilize the system. We also demonstrate that the CNT network is active in switching the devices back to the HRS, different than how other metals interact and affect the switching mechanisms in RRAM [5] , [6] . Finally, we simulate the I-V characteristics and temperature of the device in a self-consistent manner, and we determine that both the initial breakdown of the CNTs and the switching from a LRS to a HRS is thermally driven. These calculations suggest that the primary switching mechanism from the LRS to the HRS is through oxidation. Initial breakdown of carbon nanotube networks We make I-V sweeps in Fig. 1a of two-terminal devices until their current drops suddenly, indicating a physical breakdown of the device. Devices were fabricated using a dip-coating method to deposit a very dense network of CNTs on top of thermally grown SiO 2 (see Methods section for additional details) [19] , [20] . The average length of an individual CNT in our network is ~0.5 μm, shorter than our smallest devices (length~1.2 μm). An atomic force microscope (AFM) image of a CNT network device before and after breakdown in Fig. 1b,c , respectively, shows the formation of a nanometer-sized gap in the network. While the gap distance within an individual CNT network may vary from ~10 to 40 nm, similar to individual CNTs [14] , [15] , the average gap distance along the network is typically ~15 nm, with a variation of ±3 nm between devices. We also note that the gap region is mostly uniform, but may contain a small region where the gap is much larger (such as the right part of Fig. 1c ). Typically the uniform region of the nano-gap varies by <±5 nm. It is in this uniform region of the nano-gap that the following results and discussion are relevant. To lower the chances of premature breakdown from oxidation, all measurements are performed in vacuum (10 −5 Torr). It is interesting to note that for the majority of our devices, AFM could not detect any change in the surface morphology of the SiO 2 immediately following breakdown of the CNTs. This is unlike previous reports regarding Joule breakdown of individual CNTs and graphene in vacuum [12] , [15] , suggesting that the energy that would normally go towards melting the SiO 2 is being dissipated very efficiently throughout the network. 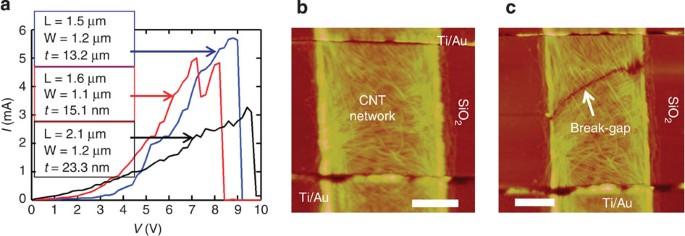Figure 1:I-Vbreakdown curves and atomic force microscopy images. (a) Examples of three differentI-Vbreakdown curves of carbon nanotube (CNT) network devices operating in vacuum. Dimensions of the length (L), width (W) and thickness (t) of each device are listed (b) Atomic force microscopy image of an as-deposited CNT network device. (c) The same CNT network device as in (b) after breaking. Scale bar, 0.5 μm. Figure 1: I-V breakdown curves and atomic force microscopy images. ( a ) Examples of three different I-V breakdown curves of carbon nanotube (CNT) network devices operating in vacuum. Dimensions of the length (L), width (W) and thickness ( t ) of each device are listed ( b ) Atomic force microscopy image of an as-deposited CNT network device. ( c ) The same CNT network device as in ( b ) after breaking. Scale bar, 0.5 μm. Full size image After the initial breakdown of the network, we observe an unusually strong coalescence induced mode (CIM) at ~1,860 cm −1 in the Raman spectrum, shown in Fig. 2a . The CIM peak is characteristic of linear sp hybridized carbon chains associated with the coalescence of adjacent CNTs [21] , [22] . We note previous studies report coalescence temperatures ranging from ~1,200–1,600 °C (refs 21 , 22 , 23 ). Spatial Raman mapping of the ratio of the CIM peak intensity to the G-peak intensity, I CIM /I G , reveals that the CIM peak is localized around the break-gap in Fig. 2b . This location is where the temperature of the CNT network is the hottest at the moment just before breaking, understanding that the breakdown process is caused by thermal stress. Therefore, it seems as if broken CNTs begin to coalesce at roughly ~1,500 °C, slightly lower than other breakdown temperatures reported for sp 2 hybridized carbon allotropes in an oxygen-depleted environment [15] , [24] . From Raman spectra, we observe that the CIM peak frequency is greater than the G-peak frequency, implying that the linear carbon chains have a higher Debye energy than the CNTs, as these Raman peaks set the approximate value of the Debye energy. Therefore, we propose that, when the CNTs break under vacuum, their Debye energy is reached and thus they become unstable and break. However, as the Debye energy for linear carbon chains is higher, they can still be formed without breaking. Namely, the unusually intensive CIM peak intensity confirms our interpretations. Fusing of CNTs is what minimizes sample to sample variation in gap size, important for consistent device performance. Nanotube coalescence is likely important for diverting energy that would otherwise go towards melting the underlying substrate. By contrast, the same experiment performed by biasing palladium lines (the same dimensions as our CNT strips) up to breakdown showed both larger gap sizes as well as larger variations in gap sizes (see Methods and Supplementary Fig. 1 ). 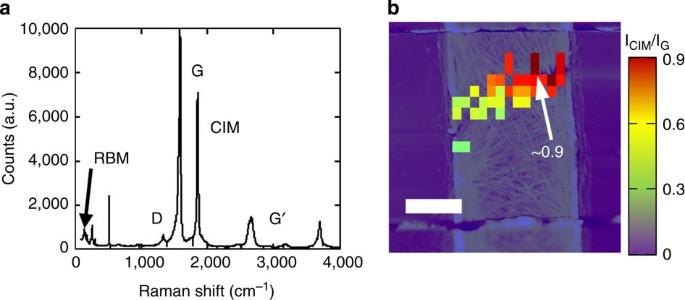Figure 2: Raman spectrum of a broken carbon nanotube network device. (a) The coalescence-induced mode (CIM) peak is most prevalent after the initial breakdown of the device. (b) Raman mapping of theICIM/IGratio of a broken device. The CIM peak is observed predominantly around the break-gap region. The darkest red represents the maximum intensity ratio ofICIM/IG~0.9, while the purple background represents a ratio of 0. Scale bar, 0.5 μm. Figure 2: Raman spectrum of a broken carbon nanotube network device. ( a ) The coalescence-induced mode (CIM) peak is most prevalent after the initial breakdown of the device. ( b ) Raman mapping of the I CIM /I G ratio of a broken device. The CIM peak is observed predominantly around the break-gap region. The darkest red represents the maximum intensity ratio of I CIM /I G ~0.9, while the purple background represents a ratio of 0. Scale bar, 0.5 μm. Full size image Switching behaviour After breaking the CNT network, we sweep the voltage back to zero, as shown in Fig. 3a . At some voltage V LRS the current increases very suddenly and sets the system in a LRS. After a LRS is recovered, we can achieve a HRS simply by increasing the biased voltage until the current drops suddenly again at V HRS . We always find that V HRS always occurs at higher voltages than V LRS . As Fig. 3a demonstrates, the device exhibits unipolar switching behaviour (for example, switching behaviour does not depend on the applied bias polarity). We can reliably switch the device multiple times between HRS and LRS. 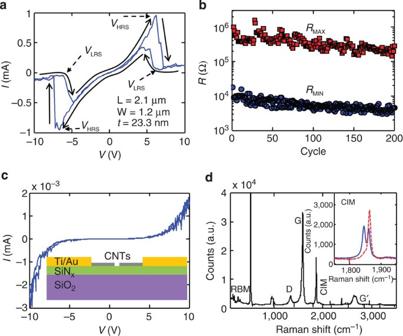Figure 3: RepresentativeI-Vcycling curve after breaking the device. (a) Sweeping downward from high-bias, the device switches to a low resistive stateatVLRS. The device breaks again and returns to its high-resistive state atVHRS. (b) The maximum and minimum resistance values in each cycle. Each time the device cycles, the resistance changes by ~ × 100. Over time, both resistance values drift to lower values. (c)I-Vcurve of a broken device fabricated on top of 100 nm of SiNx(schematic shown in the inset). The device is no longer able to switch. (d) Raman spectra of the device on SiNxafter attempting to cycle the device. (Inset) Comparison of the coalescence induced mode (CIM) peak of a device after the initial breakdown on SiNx(solid blue line) and after one cycle (red dashed line), showing that the CIM peak does not diminish when no switching events occur. Figure 3b demonstrates up to 200 switching cycles between a HRS, extracted as the maximum resistance in one cycle R MAX , and a LRS, extracted as the minimum resistance in one cycle R MIN . Over time, we observe that both the R MAX and R MIN drift to lower resistance values with approximately the same slope. After 200 cycles, we observe physical degradation of the substrate. It is possible that this drift was encountered because we were sweeping the voltage, thereby adding unnecessary electrical and thermal stress to the devices during testing. To avoid overstressing the device and to improve the reliability, we should switch the devices using short voltage pulses. Interestingly, the CIM peak height also decreases as we continue to cycle our device, indicating that the CNT network is also undergoing physical changes. Figure 3: Representative I-V cycling curve after breaking the device. ( a ) Sweeping downward from high-bias, the device switches to a low resistive stateat V LRS . The device breaks again and returns to its high-resistive state at V HRS . ( b ) The maximum and minimum resistance values in each cycle. Each time the device cycles, the resistance changes by ~ × 100. Over time, both resistance values drift to lower values. ( c ) I-V curve of a broken device fabricated on top of 100 nm of SiN x (schematic shown in the inset). The device is no longer able to switch. ( d ) Raman spectra of the device on SiN x after attempting to cycle the device. (Inset) Comparison of the coalescence induced mode (CIM) peak of a device after the initial breakdown on SiN x (solid blue line) and after one cycle (red dashed line), showing that the CIM peak does not diminish when no switching events occur. Full size image To prove that the conductive filament reconnecting the broken CNT network forms through the SiO 2 substrate, we fabricated devices where we deposit a 100 nm film of SiN x between the CNTs and SiO 2 . Figure 3c shows that we get no switching, and we can only detect a very small microampere leakage current. Therefore, just as ref. 10 had shown, switching occurs through the SiO 2 and not through the nanotubes by reconnecting through linear carbon chains or other carbon nanostructures [25] . Similar to the devices where the CNT networks are directly on top of the SiO 2 , we observe a CIM mode in the Raman spectra of CNTs on SiN x after the initial breaking of the CNT network, confirming the network stabilization through carbon linear chain formation as stated above. However, unlike the behaviour of devices directly on top of SiO 2 , the application of a high bias after breaking the SiN x -based devices does not diminish the intensity of the CIM peak, as can be seen in the inset of Fig. 3d . Furthermore, when we replaced the CNT network with Pd strips directly on SiO 2 , we were able to observe switching behaviour (see Methods and Supplementary Fig. 1b ). However, the switching voltages of these device switches varied greatly from cycle to cycle, possibly from the continued electromigration of Pd under high electric fields. As we noticed that the CIM peak decreases with each cycle, we hypothesize that the CNTs contribute to the switching behaviour of the device. While the mechanism for creating a LRS is well understood [10] , [11] , it is not clear what mechanism is responsible for returning the device to a HRS. Previous in-situ TEM measurements show that after switching to a HRS, the nano-crystal Si filament shrinks but is still present [11] . Consistent with previous work from refs 10 , 18 , the switching behaviour is unipolar with V HRS greater than V LRS , unlike conventional unipolar RRAM switching behaviour. The unipolar switching nature of the devices indicates that a thermal stress is inducing the HRS. As the initial breakdown of the CNT network happens through thermal stress, we first compare the breakdown power P BD of the CNT network with the subsequent breakdown power at V HRS in Fig. 4a , comparing devices of the same dimensions (See Supplementary Fig. 2 and Supplementary Note 1 ). We observe that all subsequent breakdowns at V HRS occur at powers that are an order magnitude lower than the initial breakdown, indicating that switching to a HRS occurs at a much lower temperature. To get an idea of what that temperature might be, and to further investigate the breakdown mechanism, we employ a two-dimensional finite element thermal model where we take into account both thermal generation by Joule heating and thermal dissipation through the electrical contacts and the underlying substrate. 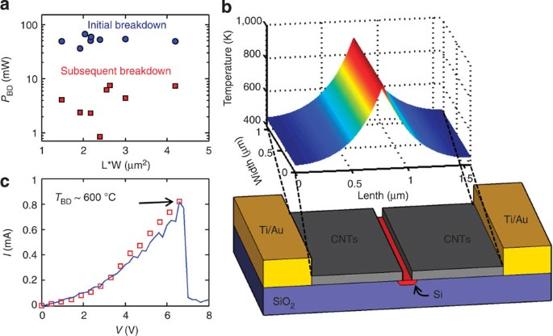Figure 4: Thermal simulation results. (a) Comparison across eight different devices showing that the initial breakdown power of the as-deposited devices is much higher than subsequent breakdowns of the CNT-SiO2-CNT device, thereby indicating a different breaking mechanism. (b) Simulated temperature profile of the same device at breakdown shown over a schematic of the device geometry used in the model. (c) BreakdownI-Vcurve of a CNT-SiO2-CNT device. The solid line represents raw data and the symbols represent the simulatedI-Vcurve up to breakdown. Figure 4: Thermal simulation results. ( a ) Comparison across eight different devices showing that the initial breakdown power of the as-deposited devices is much higher than subsequent breakdowns of the CNT-SiO 2 -CNT device, thereby indicating a different breaking mechanism. ( b ) Simulated temperature profile of the same device at breakdown shown over a schematic of the device geometry used in the model. ( c ) Breakdown I-V curve of a CNT-SiO 2 -CNT device. The solid line represents raw data and the symbols represent the simulated I-V curve up to breakdown. Full size image Similar to previous reports, we integrate our thermal model (see Methods and Supplementary Fig. 3 ) into our I-V curve simulation by self-consistently calculating the current output and temperature of our device [14] , [15] , [26] , [27] . To calculate the temperature of the device, we use finite element modelling of the two-dimensional heat transport equation where κ is the thermal conductivity of the CNT network, T is the device temperature, T 0 is the ambient temperature, G is the heat loss into the substrate, V is the volume and P is the power generated through Joule heating ( P=I 2 R ). To account for heat dissipation into the underlying substrate, we rely on previously extracted thermal resistance values and shape factors for CNTs and CNT networks on SiO 2 (refs 14 , 15 , 28 , 29 , 30 ). To calibrate our thermal model, we first simulate a device before breaking the CNT network. By matching the calculated I-V curve to raw data (shown in Supplementary Fig. 3 ) and setting the breakdown temperature to be 2,301.3 K (which is the temperature associated with the G-band zone-centre phonon; an approximation for the Debye temperature of the CNT networks), we can extract the relationship between the resistivity and temperature for each device. Each device generates a unique resistivity dependence on temperature because the thermal properties of CNT networks [31] vary depending on nanotube diameter, chirality and metalicity. The ability to experimentally capture the temperature dependence on the resistivity of each individual device negates the need to know accurately how these variations impact heat generation and dissipation in CNT networks. Measuring the temperature dependence also removes the need to model non-equilibrium effects (for example, hot electrons), which may be present in our experiments. We use the extracted temperature dependence of the resistivity of the CNT network in the simulation of the device schematic depicted in the bottom of Fig. 4b . The simulated temperature profile shown in the top of Fig. 4b indicates that the filament is the hottest when the device is biased at V HRS . Not included in our simulation are localized hotspots within the CNT network caused by spatial density variations within the network [28] , [29] . The temperature rise at these local hotspots are small when compared with the average temperature rise of the device. Even when the filament is moved closer to one of the contacts, we calculate that the maximum temperature of the device is still in the filament. We simulate the I-V curve of a device up to its switching voltage, shown in Fig. 4c . We note that we can reproduce our data quite accurately using temperature to determine the resistivity of the sample. If, instead of calibrating with temperature, we calibrate the resistivity of the CNT network using the applied bias from the initial breakdown curve, we are not able to reproduce the I-V characteristics of the CNT-Si-CNT device. Therefore, we emphasize that the switching to the HRS must be through a thermally induced process and is not driven by the applied electrical field. From the simulation, we can associate a breakdown temperature, T BD with V HRS , which from Fig. 4c , occurs at ~600 °C±100 °C. This switching temperature also happens to be the oxidation temperature of CNTs [15] , [27] , [32] . Previously, CIM peaks have only been reported when CNTs reach ~1,500 °C in a vacuum environment. However, our thermal simulation suggests that the switches are only able to sustain temperatures up to ~600 °C. We recall from our Raman measurements that after cycling the device, the intensity of the CIM peak decreases. The decrease in intensity suggests that we are not forming CIM modes anymore, but rather decreasing their occurrence. Therefore, combining evidence from Raman spectroscopy together with our simulations suggests that the CNTs are slowly oxidizing or are interacting with oxygen atoms to break contact to the conductive filament. The repeated oxidation of the CNTs may also play a role in the drift of R MAX and R MIN observed in Fig. 3b , by very slowly increasing the size of the filament. As all measurements in this study are performed in a vacuum environment, the most likely source of oxygen comes from the SiO 2 itself. When the applied fields and temperatures are high, oxygen ions may propagate through or around the filament to the CNT networks. Previous systems that exhibit bipolar switching behaviour (dependence on positive or negative polarity) have attributed the bipolar switching nature to the partial oxidation of the metal contacts [6] , [33] . However, in this case unipolar switching behaviour is observed because electrical contact is not broken until the CNTs undergo oxidation. Finally, we rule out amorphization of the Si nano-crystals as a switching mechanism [11] . The measurements in this study were performed using continuous voltage sweeps rather than pulsed voltages. Therefore, no thermal quenching condition could possibly be achieved through our measurements. In conclusion we used dense CNT networks as contact electrode materials for a MIM switch. Using CNT networks allows controllability over the placement of CNTs, a necessity for scaling fabrication up to wafer level. We show that during the breakdown of a CNT network, individual CNTs stabilize themselves shortly after breakdown by coalescing with neighbouring CNTs, forming linear chains. After forming the conductive filament to make the MIM switch, the breakdown mechanism becomes substrate-induced oxidation. This new switching mechanism, together with the robustness of Si, leads to V HRS > V LRS , removing the need to set current limits. In addition to being used for NVM technology, these devices could be used in field programmable arrays as fuses and anti-fuses. As an LRS state can be recovered, it is also conceivable that failure of any electrically contacted CNT network device (that is, transistors and interconnects) surrounded by SiO 2 could be recovered, albeit with decreased performance. Device fabrication First, silicon wafers were thermally oxidized to grow a high quality layer of SiO 2 . We did not dope the SiO 2 with any metallic impurities. The surface of the SiO 2 was then treated using a plasma process to improve the dip-coating deposition of CNTs to the substrate [19] , [20] . A layer of polymethyl methacrylate was then patterned with electron beam lithography to define windows where CNTs were to be deposited on the surface. We then deposit CNTs by either pulling the substrate very slowly out of a solution of CNTs dispersed in deionized water, or simply by letting the solution evaporate while the substrate is oriented perpendicular to the liquid surface. The meniscus forces push the CNTs onto the surface and offer a small degree of alignment with the pulling direction. We then lift off the undesired CNTs leaving only strips of CNT networks shown in Fig. 1a,b . We use the same lithography and lift-off process for defining electron beam evaporated contacts. Palladium-Si-Palladium control As a control experiment, we made contacts with thin palladium strips with the same dimensions and geometry as the devices with a CNT network channel, as shown in the optical micrograph image in Supplementary Fig. 1a . We apply a bias across the Pd strip until it breaks. The break-gap created in the Pd strip is very large (several micrometres) when compared with the break-gap in the CNT network devices (several nanometers). We are able to still observe the same general switching behaviour in the Pd strip as in the CNT-Si-CNT devices. The I-V curve for a Pd-Si-Pd device is shown in Supplementary Fig. 1b . We note that the current after numerous switches to a HRS is unstable and sometimes briefly switches back to the LRS. Therefore, while CNTs are not necessary to achieve switching behaviour, they are important for achieving consistent operating performance in a planar device. Temperature-dependent I-V calculations We calculate the I-V curves and temperature profile of the devices in a self-consistent manner. To calculate the temperature of a device, we discretize the Equation (1) and solve it using an iterative successive over relaxation scheme. We assume an anisotropic thermal conductivity for the CNT network, where the thermal conductivity along the length of the CNT network (running from one electrical contact to the other) is 50 W m −1 K −1 , and 20 W m −1 K −1 for the perpendicular thermal conductivity [31] . However, it turns out that our calculations were not very sensitive to the thermal conductivity and values up to 300 W m −1 K −1 resulted in <3% change in calculated temperature for most devices, as most of the heat gets dissipated into the underlying substrate. We use 1.2 × 10 7 K −1 W −1 for the thermal resistance of the CNT-metal boundary [27] . We assume that no heat is transported from the CNT to the vacuum environment. We treat the heat loss into the substrate as heat being emitted from a rectangular slab, which is calculated from the following expression [34] : where L is the length of the CNT network (distance between electrodes), t ox is the oxide thickness, W is the width of the CNT network (perpendicular to the length and in the plane of the CNT network), κ ox is the thermal conductivity of the oxide and R Cox is the thermal resistance of the CNT/SiO 2 interface (1 × 10 −8 m 2 K W −1 ). The first term in Equation (2) accounts for 3-D heat spreading into the underlying substrate. Next we use the raw I-V breakdown curve of a pristine device, shown in Supplementary Fig. 3a , to input the breakdown power of the CNTs into our model. We set the breakdown temperature, T BD =2,301.3 K, the temperature associated with the zone-centre phonon energy that gives rise to the G-band peak. The only parameter that is now unknown is the contact resistance of the device. We modulate the contact resistance until we are able to match the breakdown power with the correct T BD . We match T BD to the maximum temperature of the calculated temperature profile of the unbroken CNT shown in Supplementary Fig. 3b . After extracting the contact resistance, we input the power at different biases from Supplementary Fig. 3a to calculate a corresponding temperature for the device, thus extracting the temperature dependence of the CNT network resistivity. We input this result into our simulation of the CNT-Si-CNT device, and calculate the I-V curve from the resistivity of the CNT, along with the device temperature in a self-consistent manner. We do not modulate the Si resistivity with temperature. As the Si filament is only ~15 nm and consists of smaller nano-crystallites, it is likely that electron conduction between grains is ballistic, and should therefore have little dependence on temperature. We modulate the Si resistivity to get quantitative matching between our measured and simulated I-V curves. Similar to ref. 10 , we extract a resistivity of ~10 −2 −10 −3 Ω-cm, when using the entire width of the nano-gap. Without the temperature-dependent CNT resistivity, however, we are not able to even qualitatively fit our data. How to cite this article : Liao, A. D. et al. Carbon nanotube network-silicon oxide non-volatile switches. Nat. Commun. 5:5673 doi: 10.1038/ncomms6673 (2014).